Energy-filtered cold electron transport at room temperature Fermi-Dirac electron thermal excitation is an intrinsic phenomenon that limits functionality of various electron systems. Efforts to manipulate electron thermal excitation have been successful when the entire system is cooled to cryogenic temperatures, typically <1 K. Here we show that electron thermal excitation can be effectively suppressed at room temperature, and energy-suppressed electrons, whose energy distribution corresponds to an effective electron temperature of ~45 K, can be transported throughout device components without external cooling. This is accomplished using a discrete level of a quantum well, which filters out thermally excited electrons and permits only energy-suppressed electrons to participate in electron transport. The quantum well (~2 nm of Cr 2 O 3 ) is formed between source (Cr) and tunnelling barrier (SiO 2 ) in a double-barrier-tunnelling-junction structure having a quantum dot as the central island. Cold electron transport is detected from extremely narrow differential conductance peaks in electron tunnelling through CdSe quantum dots, with full widths at half maximum of only ~15 mV at room temperature. At finite temperatures, electrons in solids are thermally excited in accordance with the Fermi-Dirac distribution. This electron thermal excitation obscures or nullifies many novel and technologically important phenomena in various electron systems. For example, it can wipe out the Coulomb blockade in single-electron systems [1] , [2] , [3] and deteriorate the efficiency of spin-valve effect in spintronic systems [4] , [5] , [6] . Electron thermal excitation can also significantly degrade the performance of more mainstream electronic devices. For example, it is the root cause of excessive power dissipation in complementary metal-oxide-semiconductor (CMOS) transistors [7] , [8] . These are just a few examples, but the negative effect of electron thermal excitation prevails in solid-state electron systems in general. Therefore, if there were a method that could enable manipulation of electron thermal excitation, a broad range of scientific and technological benefits would be expected. Previous studies by others have demonstrated that it is possible to suppress electron thermal excitations, and thereby obtain low-temperature electrons, by utilizing discrete energy levels present in quantum dots (QDs) [9] , [10] , [11] . If electron transport is made to occur through a discrete energy level, it can serve as an energy filter (or thermal filter) as only those electrons whose energies match the discrete energy level are allowed to participate in the transport. This has been experimentally demonstrated using double QD systems, in which the first QD adjacent to the source electrode serves as an energy filter, passing only cold electrons to the second QD [9] , [10] , [11] . In a similar manner, it has also been demonstrated that the discrete energy levels or superconducting energy gaps can be utilized for quantum cooling of electron gases through energy-selective electron tunnelling [12] , [13] , [14] , [15] , [16] . Until now, studies have been focused on obtaining ultralow sub-Kelvin electrons and investigating their novel phenomena when the entire system is cooled to cryogenic temperatures, typically less than 1 K (refs 9 , 10 , 11 , 12 , 13 , 14 , 15 , 16 ). In this work, we focus the study on much higher temperature regime, the room temperature. We show that electron thermal excitation can be effectively suppressed at room temperature and the energy-suppressed electrons, whose energy distribution corresponds to an effective electron temperature of ~45 K, can be transported throughout device components without any external cooling. This is demonstrated using a structure having a sequential arrangement of a source electrode, a quantum well (QW), a QD and a drain electrode, in which a discrete state of the QW serves as an energy filter as electrons are transported from the source to the drain. The key aspect of this approach is that once electrons are filtered by the QW state, they cannot gain energy because no path exists for electron excitation (except for the phonon absorption that we will discuss later), and therefore, the electrons remain cold until transported to the drain. This approach can be used as an effective strategy to circumvent the intrinsic thermodynamic constraint of electron thermal excitation and may lead to many practical applications. An example is demonstrated using single-electron transistors (SETs), in which the use of energy-filtered cold electrons eliminates the need of liquid He cooling and produces Coulomb staircase and Coulomb oscillations at room temperature. Cold electron transport at room temperature We created an energy filtering structure by incorporating a QW into a double-barrier tunnelling junction (DBTJ) configuration, Fig. 1a . When a voltage bias is applied to the usual DBTJ such that an energy level of the QD ε D is brought close to the Fermi level μ L of the source electrode ( Fig. 1a left), electrons can tunnel from the source to the QD, resulting in a current onset in the I – V characteristics ( Fig. 1a bottom left). At finite temperatures, however, this current onset is not abrupt because thermally excited electrons in the source electrode can tunnel to the QD even if ε D is positioned above μ L (red arrow in Fig. 1a left). This situation changes dramatically if we insert a QW between the source and tunnelling barrier 1 ( Fig. 1a right). In this case, the electron transport from the QW energy level ε W to the QD energy level ε D can occur only if ε D is equal to or lower than ε W (red arrow in Fig. 1a right) [17] . If ε D is positioned above ε W , the transport will be blocked as there is no available excitation path (except for the phonon absorption that can occur when the energy level offset is small, which we will discuss later). This will produce an abrupt current step where the current onset corresponds to the alignment of ε W and ε D ( Fig. 1a bottom right). 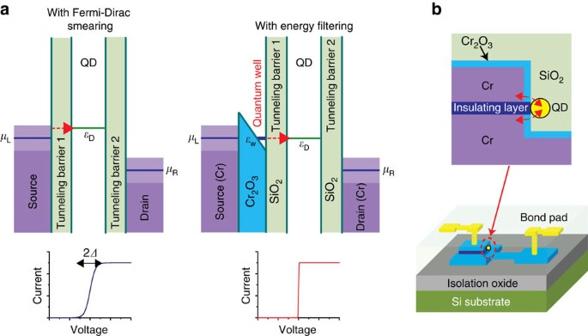Figure 1: Schematic of electron energy filtering for cold electron transport. (a) Left: the double-barrier tunnel junction (DBTJ) structure. Due to the Fermi-Dirac thermal excitation, electron tunnelling can occur (red arrow) even if QD energy levelεDis not perfectly aligned with the source Fermi levelμL, resulting in broadened current onset in theI–V, bottom left. The broadening Δ of the current step increases with temperature. The light-coloured shades near the Fermi levelsμLandμRschematically represent the Fermi-Dirac thermal smearing in the electrodes. (a) Right: DBTJ structure with a quantum well inserted between the source and tunnelling barrier 1. A discrete energy level formed in the QW serves as an energy filter for electron injection to the QD. The current onset occurs when the QD energy levelεDaligns with the QW energy levelεW, resulting in a sharp current jump in theI–V, bottom right. The QW formed on the drain side does not contribute to the energy filtering, as under the conditionεD>μR, electrons in the QD will tunnel out to the drain anyway without regard to the presence of QW in the drain side. For simplicity, the schematic does not include the QW on the drain side. (b) Schematic of the DBTJ structure with the energy filter inserted. Top: cross-sectional view. The dotted arrows indicate electron tunnelling paths. Bottom: three-dimensional view of one device unit. The schematics are not to scale. Figure 1: Schematic of electron energy filtering for cold electron transport. ( a ) Left: the double-barrier tunnel junction (DBTJ) structure. Due to the Fermi-Dirac thermal excitation, electron tunnelling can occur (red arrow) even if QD energy level ε D is not perfectly aligned with the source Fermi level μ L , resulting in broadened current onset in the I – V , bottom left. The broadening Δ of the current step increases with temperature. The light-coloured shades near the Fermi levels μ L and μ R schematically represent the Fermi-Dirac thermal smearing in the electrodes. ( a ) Right: DBTJ structure with a quantum well inserted between the source and tunnelling barrier 1. A discrete energy level formed in the QW serves as an energy filter for electron injection to the QD. The current onset occurs when the QD energy level ε D aligns with the QW energy level ε W , resulting in a sharp current jump in the I – V , bottom right. The QW formed on the drain side does not contribute to the energy filtering, as under the condition ε D > μ R , electrons in the QD will tunnel out to the drain anyway without regard to the presence of QW in the drain side. For simplicity, the schematic does not include the QW on the drain side. ( b ) Schematic of the DBTJ structure with the energy filter inserted. Top: cross-sectional view. The dotted arrows indicate electron tunnelling paths. Bottom: three-dimensional view of one device unit. The schematics are not to scale. Full size image We formed the QW between the source and tunnelling barrier 1 (SiO 2 ) by using Cr as the source electrode, for which a thin layer (~2 nm) of Cr 2 O 3 is naturally formed on the Cr surface and serves as the QW material ( Fig. 1a right). Here the interface charges and/or interface dipoles at the Cr 2 O 3 /SiO 2 interface [18] , [19] , [20] , [21] induce a band bending of the Cr 2 O 3 conduction band, producing the QW [22] , [23] , [24] , [25] , [26] (the measured depth of the QW: 1.1±0.1 eV; see Supplementary Figs 1 and 2 and Supplementary Note 1 ). We fabricated this energy structure in a three-dimensional configuration using the procedure previously reported [27] ( Fig. 1b ). In this configuration, the electrodes (Cr) are vertically separated by an insulating layer (SiO 2 or Al 2 O 3 ), the QD is positioned at the sidewall of the insulating layer, and the SiO 2 between the QD and electrode serves as the tunnelling barrier. We used CdSe nanoparticles as QDs and investigated the electron transport through their discrete energy states. 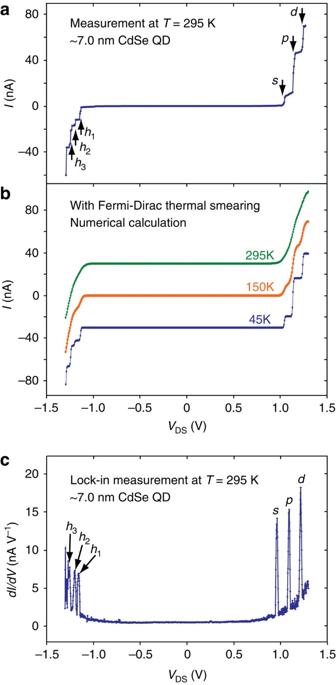Figure 2: Demonstration of energy-filtered cold electron transport at room temperature. (a)I–Vcharacteristics measured at room temperature. The unit was fabricated with the structure inFig. 1band with ~7.0-nm CdSe nanocrystal (nominal size) as the QD. Arrows indicate abrupt current jumps. Each current jump corresponds to an alignment of the QW levelεWto a discrete energy level of the CdSe QD. (b) Numerically calculatedI–V’s under the usual Fermi-Dirac smearing (no energy filtering) at different temperatures (simulator: SIMON 2.0). TheI–Vat 45 K reproduces the room temperature experimental data ina. At room temperature, the current steps are wiped out due to Fermi-Dirac thermal smearing. TheI–V’s are vertically displaced by 30 nA for clarity. (c) Direct differential conductance (dI/dV) measurement using the lock-in technique at room temperature (the measurements inaandcare from different units). The peaks resulted from the alignment of the QW levelεWto discrete energy levels of the CdSe QD. The peak widths are extremely narrow even at room temperature: their full widths at half maximum (FWHMs) are ~18 mV.s,p,dandh1,h2,h3: the first three QD levels in the conduction and valence band, respectively. Figure 2a shows the I – V characteristics measured at room temperature for a unit in which a ~7 nm CdSe nanoparticle was used as the QD. Abrupt current jumps (indicated by arrows) are clearly resolved, which reveals that the energy filtering and subsequent cold electron transport work extremely well at room temperature. Each current jump corresponds to the alignment of an energy level of the CdSe QD with the QW energy level ε W , where s , p and d represent the first three levels in the conduction band of the CdSe QD and h 1 , h 2 and h 3 the first three levels in the valance band. We also see a clear zero-conductance gap (~2.2 V), which originates from the band gap of the CdSe QD. Figure 2: Demonstration of energy-filtered cold electron transport at room temperature. ( a ) I – V characteristics measured at room temperature. The unit was fabricated with the structure in Fig. 1b and with ~7.0-nm CdSe nanocrystal (nominal size) as the QD. Arrows indicate abrupt current jumps. Each current jump corresponds to an alignment of the QW level ε W to a discrete energy level of the CdSe QD. ( b ) Numerically calculated I – V ’s under the usual Fermi-Dirac smearing (no energy filtering) at different temperatures (simulator: SIMON 2.0). The I – V at 45 K reproduces the room temperature experimental data in a . At room temperature, the current steps are wiped out due to Fermi-Dirac thermal smearing. The I – V ’s are vertically displaced by 30 nA for clarity. ( c ) Direct differential conductance (d I /d V ) measurement using the lock-in technique at room temperature (the measurements in a and c are from different units). The peaks resulted from the alignment of the QW level ε W to discrete energy levels of the CdSe QD. The peak widths are extremely narrow even at room temperature: their full widths at half maximum (FWHMs) are ~18 mV. s , p , d and h 1 , h 2 , h 3 : the first three QD levels in the conduction and valence band, respectively. Full size image For electron transport without the energy filtering, abrupt current steps can be obtained only at low temperatures. Figure 2b shows numerically calculated I – V ’s at varying temperatures in which the Fermi-Dirac thermal excitation governs their temperature behaviour. We see that the experimental I – V in Fig. 2a can be achieved only when the temperature is brought to ~45 K (blue in Fig. 2b ), where thermal excitation is sufficiently suppressed. At room temperature, all the current steps are wiped out because of Fermi-Dirac thermal excitation (green in Fig. 2b ). Experimentally, electron transport through a QD in the usual DBTJ was extensively studied by others using scanning tunnelling spectroscopy (STS) [28] , [29] , [30] , [31] , [32] . We note that their well-resolved current steps were observed only at low temperatures (<5 K), most often accompanied by non-thermal broadening factors, such as optical phonon contributions [28] , [29] , [30] , [31] , [32] , [33] , [34] , [35] . For example, the I – V characteristics obtained for a CdSe QD showed that the broadening Δ (definition in Fig. 1a ) is ~50 mV at 4.5 K (ref. 31 ). On the other hand, our method led to much more abrupt current steps even at room temperature; Δ is only ~20 mV at 295 K ( Fig. 2a ). To further investigate the abrupt current jumps in Fig. 2a , we carried out independent direct differential conductance (d I /d V ) measurements using the lock-in technique at room temperature ( Fig. 2c; the data in Fig. 2a, c are from different units). We observe well-resolved peaks, each corresponding to the current step in the I – V measurement in Fig. 2a . The peak widths in Fig. 2c are extremely narrow; the full widths at half maximum (FWHMs) of the peaks are only ~18 mV. 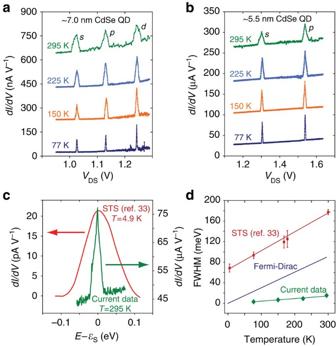Figure 3: Effectiveness of the energy filtering manifested in narrow dI/dVpeak widths at different temperatures. (a) dI/dV’s at different temperatures for ~7.0 nm CdSe QD. The first three energy levels (labelled ass,pandd) in the QD conduction band are shown. (b) dI/dV’s at different temperatures for ~5.5 nm CdSe QD. The first two energy levels (sandp) in the QD conduction band are shown. Note that the voltage scales are different foraandb. For each measurement inaandb, there was a slight shift of peak positions (<15 mV) because of the background charge3,31(the relative peak separations remained the same). We have shifted the peak positions so that all thespeaks are aligned to thespeak of 77 K. The 7.0 nm and 5.5 nm inaandbare the nominal diameters of the CdSe QD colloids. (c) Comparison of the peak widths. Green: room temperature measurement from this study (thespeak at 295 K inb). Red: STS measurement of a CdSe QD at 4.9 K by Jdiraet al.33E: electron energy;εs: energy of QDs-level. (d) FWHMs of the dI/dVpeaks at different temperatures. Red: STS measurements by Jdiraet al.33; the error bars represent standard deviations of the FWHMs from several CdSe QDs. Blue: calculation with the usual Fermi-Dirac thermal smearing (Supplementary Note 5). Green: current experiment. Forcandd, the energy scale (eV or meV) is used, for which the voltage divisions across the tunnelling junctions 1 and 2 have been taken into account (Supplementary Notes 3 and 4). Were the usual Fermi-Dirac thermal smearing in effect, the same FWHMs could have been obtained only when the temperature were lowered to ~45 K. Temperature dependance To investigate the effect of temperature on the energy filtering, we carried out differential conductance measurements (using lock-in) at varying reservoir temperatures, ranging from 77 to 295 K. Figure 3a displays differential conductances obtained from a unit in which an ~7-nm CdSe nanoparticle was used as the QD. We find that the peak widths decrease as the temperature is lowered; the FWHMs are ~16, ~10, ~7 and ~3 mV at 295, 225, 150 and 77 K, respectively. At each temperature, the peak widths are the same for all s , p and d peaks. Figure 3: Effectiveness of the energy filtering manifested in narrow d I /d V peak widths at different temperatures. ( a ) d I /d V ’s at different temperatures for ~7.0 nm CdSe QD. The first three energy levels (labelled as s , p and d ) in the QD conduction band are shown. ( b ) d I /d V ’s at different temperatures for ~5.5 nm CdSe QD. The first two energy levels ( s and p ) in the QD conduction band are shown. Note that the voltage scales are different for a and b . For each measurement in a and b , there was a slight shift of peak positions (<15 mV) because of the background charge [3] , [31] (the relative peak separations remained the same). We have shifted the peak positions so that all the s peaks are aligned to the s peak of 77 K. The 7.0 nm and 5.5 nm in a and b are the nominal diameters of the CdSe QD colloids. ( c ) Comparison of the peak widths. Green: room temperature measurement from this study (the s peak at 295 K in b ). Red: STS measurement of a CdSe QD at 4.9 K by Jdira et al . [33] E : electron energy; ε s : energy of QD s -level. ( d ) FWHMs of the d I /d V peaks at different temperatures. Red: STS measurements by Jdira et al . [33] ; the error bars represent standard deviations of the FWHMs from several CdSe QDs. Blue: calculation with the usual Fermi-Dirac thermal smearing ( Supplementary Note 5 ). Green: current experiment. For c and d , the energy scale (eV or meV) is used, for which the voltage divisions across the tunnelling junctions 1 and 2 have been taken into account ( Supplementary Notes 3 and 4 ). Full size image The small FWHMs and their temperature dependence in Fig. 3a will prevail without regard to any specific energy level of a QD as the energy filtering occurs through an energy level of the QW, not the QD. To verify this, we fabricated a unit having an ~5.5-nm CdSe QD as its central island. Differential conductance measurements at varying temperatures are shown in Fig. 3b . We find their peak positions well reflect the size dependence of QD energy levels, in agreement with the literature [30] , [36] , [37] , [38] , [39] , [40] ; compared to the unit with ~7-nm CdSe QD ( Fig. 3a ), the unit with ~5.5-nm CdSe QD shows a higher conduction band onset (at ~1.3 V) and a larger s - p level separation (~240 mV; see also Supplementary Fig. 3 and Supplementary Note 2 ). Nevertheless, the peak widths and their temperature dependence are essentially the same in Fig. 3a,b (see also Supplementary Fig. 4 , Supplementary Tables 1–3 and Supplementary Notes 3 and 4 ), demonstrating that the same energy filtering process is in effect without regard to a specific QD energy level structure. We note that the peak widths in our differential conductance measurements, in Fig. 3a,b , are much narrower than those observed by others in STS measurements of QDs in the DBTJ configuration [28] , [29] , [30] , [31] , [32] , [33] , [34] , [35] . For the latter, the FWHMs are typically larger than ~50 mV even at cryogenic temperatures (<5 K). For example, a comparison in Fig. 3c shows that the peak from room temperature measurement of this study (green) is much narrower than the one from an STS measurement of a CdSe QD at 4.9 K (red) [33] . For our experimental temperature range of 77–295 K, we find a linear relationship between the FWHMs and the temperature, which is displayed in Fig. 3d (green). The temperature dependences of the FWHMs that result from electron transport without the energy filtering are also shown in Fig. 3d , one from calculations based on Fermi-Dirac electron energy distribution (blue line; Supplementary Figs 5–7 and Supplementary Note 5 ) and the other from reported STS measurements (red) [33] . Here we note that the slope for the experimental STS data is almost the same as that from the Fermi-Dirac smearing calculations, affirming that the STS thermal behaviour is governed by the usual Fermi-Dirac smearing. Comparing all three cases in Fig. 3d , it is clear that our method has effectively filtered out hot electrons, leading to extremely narrow peak widths over all temperature ranges explored. The temperature of electrons is determined by their energy distribution [12] , [13] , which is reflected on the d I /d V peak widths. We can, therefore, obtain effective electron temperatures of the energy-filtered electrons by comparing the FWHMs of our experiment with those from the Fermi-Dirac smearing calculations. For example, at reservoir temperature of 295 K, the electron temperature becomes ~45 K; in Fig. 3d , the FWHM from Fermi-Dirac electrons at 45 K is the same as the FWHM from the energy-filtered electrons at reservoir temperature of 295 K. Likewise, we obtain electron temperatures of the energy-filtered electrons as ~35, ~22 and ~10 K for reservoir temperatures of 225, 150 and 77 K, respectively ( Supplementary Note 4 ). These cold electrons promise numerous practical applications as we will discuss in a later section. Modelling In our model, the system is made of the following components, a source (L), a QW, a QD and a drain (R), with tunnelling barriers separating them ( Fig. 4a ). We assume a one-dimensional transport model in which electrons are sequentially transported in a one-dimensional configuration space from the source to the QW, QD and drain. The transport rates between adjacent components are represented by Γ L ± ( i W ), Γ D ± ( i W ), Γ W ± ( i D ) and Γ R ± ( i D ) (see Fig. 4a for definitions). For a given set of rates (at a voltage bias V ), we simultaneously solve the rate equations [29] ( Supplementary Note 6 ), which gives an electrical current I at the bias V . 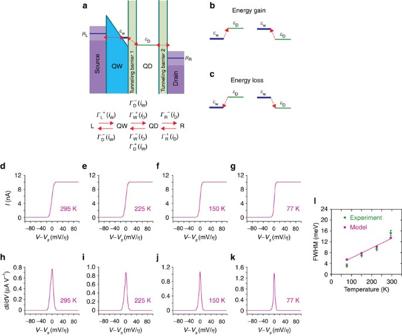Figure 4: Modelling for energy-filtered cold electron transport. (a) Energy diagram.ΓL±(iW): the rate for an electron tunnelling from the source electrode (L) to the QW (‘+’) or from QW to L (‘−’) when the number of electrons in the QWbeforethe tunnelling isiW.ΓD±(iW): the rate for an electron tunnelling from the QD to the QW (‘+’) or from QW to QD (‘−’) when the number of electrons in the QWbeforethe tunnelling isiW.ΓW±(iD): the rate for an electron tunnelling from the QW to the QD (‘+’) or from QD to QW (‘−’) when the number of electrons in the QD levelbeforethe tunnelling isiD.ΓR±(iD): the rate for an electron tunnelling from the drain electrode (R) to the QD (‘+’) or from QD to R (‘−’) when the number of electrons in the QDbeforethe tunnelling isiD. (b,c) Schematic of an inelastic tunnelling in which an electron gains (b) and loses (c) the energy, respectively. (d–g) CalculatedI–Vcharacteristics at 295, 225, 150 and 77 K, respectively.Vsis the onset voltage for tunnelling to thes-level of the QD.η: the voltage division factor (Supplementary Note 6). (h–k) Calculated dI/dV’s at 295, 225, 150 and 77 K, respectively. (l) Comparison of FWHMs of the dI/dVpeaks from the experiment (green) and model calculations (pink). The error bars represent standard deviations of the FWHMs from all peaks inFig. 3a(s,pandd) andFig. 3b(sandp) at given temperatures; see alsoSupplementary Fig. 4,Supplementary Tables 2, 3andSupplementary Note 4. Figure 4: Modelling for energy-filtered cold electron transport. ( a ) Energy diagram. Γ L ± ( i W ): the rate for an electron tunnelling from the source electrode (L) to the QW (‘+’) or from QW to L (‘−’) when the number of electrons in the QW before the tunnelling is i W . Γ D ± ( i W ): the rate for an electron tunnelling from the QD to the QW (‘+’) or from QW to QD (‘−’) when the number of electrons in the QW before the tunnelling is i W . Γ W ± ( i D ): the rate for an electron tunnelling from the QW to the QD (‘+’) or from QD to QW (‘−’) when the number of electrons in the QD level before the tunnelling is i D . Γ R ± ( i D ): the rate for an electron tunnelling from the drain electrode (R) to the QD (‘+’) or from QD to R (‘−’) when the number of electrons in the QD before the tunnelling is i D . ( b , c ) Schematic of an inelastic tunnelling in which an electron gains ( b ) and loses ( c ) the energy, respectively. ( d – g ) Calculated I – V characteristics at 295, 225, 150 and 77 K, respectively. V s is the onset voltage for tunnelling to the s -level of the QD. η : the voltage division factor ( Supplementary Note 6 ). ( h – k ) Calculated d I /d V ’s at 295, 225, 150 and 77 K, respectively. ( l ) Comparison of FWHMs of the d I /d V peaks from the experiment (green) and model calculations (pink). The error bars represent standard deviations of the FWHMs from all peaks in Fig. 3a ( s , p and d ) and Fig. 3b ( s and p ) at given temperatures; see also Supplementary Fig. 4 , Supplementary Tables 2, 3 and Supplementary Note 4 . Full size image For the electron tunnelling between the QW and the QD, we have included inelastic electron tunnelling processes. We assume that an electron tunnelling from a lower energy state to a higher energy state (energy gain) is possible if coupled with a phonon absorption [41] , [42] ( Fig. 4b ). An inelastic tunnelling from a higher energy state to a lower energy state (energy loss) occurs through phonon emission [41] , [42] and other energy relaxation processes (for example, defect-assisted relaxation, interface-roughness scattering and impurity scattering) [17] , [25] , [43] , [44] , [45] , [46] , [47] , [48] ( Fig. 4c ). With these inelastic tunnelling events taken into account, the tunnelling probabilities γ ( ε,T )’s, where ε is energy difference ( ε is defined negative when an electron gains energy and positive when loses energy) and T is the absolute temperature, are given as follows: and Here γ absorp ( ε , T ) and γ emiss ( ε , T ) are tunnelling probabilities with phonon absorption and phonon emission, respectively, and n (| ε |, T ) is the Bose–Einstein distribution function of phonon population, n ( ε , T )=1/( e ε/kT −1), where k is the Boltzmann constant. A ( ε ) is the Einstein A coefficient for spontaneous emission of phonons [41] , [42] . γ elastic ( ε ) is the elastic tunnelling probability having Lorentzian distribution [11] , [25] , [49] and γ relax ( ε ) is the tunnelling probability resulting from all other energy relaxation paths [17] , [25] , [43] , [44] , [45] , [46] , [47] , [48] ( Supplementary Note 6 ). We note that γ ( ε <0, T ) and γ ( ε >0, T ) are temperature dependent through the Bose–Einstein distribution function, which is the origin of the temperature dependence of the I – V ’s and d I /d V ’s. The tunnelling probabilities γ ( ε <0, T ) and γ ( ε >0, T ), along with the probabilities of electrons occupying the QW and QD states, determine the tunnelling rates Γ D ± ( i W ) and Γ W ± ( i D ) ( Supplementary Note 6 ). The rate equations are constructed as in equations (35)–(39) in the Supplementary Note 6 , and are solved numerically ( Supplementary Figs 8–10 and Supplementary Note 6 ). The electrical current I is then given by where e is the charge of an electron, and P D (0) and P D (1) are the probabilities that the QD is occupied by no electron and one electron, respectively. The d I /d V is obtained by numerical differentiation of the I ( V ). Figure 4d–k shows resulting I – V and d I /d V calculations at different temperatures. We find an abrupt current jump, Δ=~15 mV, at room temperature ( Fig. 4d ), in good agreement with the experimental measurement in Fig. 2a . The current jumps become more abrupt as the temperature decreases ( Fig. 4e–g ). The d I /d V ’s ( Fig. 4h–k ) show narrow peak widths, with the peak width decreasing with decreasing temperature, in good agreement with the differential conductance measurements in Fig. 3a,b . We also point out that the d I /d V peaks in Fig. 3a,b are of a triangular shape, not Gaussian or Lorentzian. Our model calculations in Fig. 4h–k faithfully reproduce the triangular-type d I /d V peaks. For quantitative comparisons, we display in Fig. 4l the FWHMs from our model calculations and those from the experimental measurements. A very good agreement is found between them over the temperature range investigated (77–295 K). Applications The electron energy filtering and its associated cold electron transport have profound technical implications. If our method can be properly implemented into an electron system/device whose operation temperature or performance is limited by the Fermi-Dirac thermal excitation, the electron energy filtering could significantly relieve those thermal limitations. Here a specific example of practical benefits of energy-filtered cold electron transport is demonstrated with SETs. We fabricated SETs using the configuration shown in Fig. 1b , but with two alterations: (i) the CdSe QD was replaced by a metal nanoparticle (~10 nm Au nanoparticle) and (ii) a gate electrode was added using the configuration reported previously, in which the gate encompasses the periphery of the source/insulating layer/drain stack in Fig. 1b [27] . 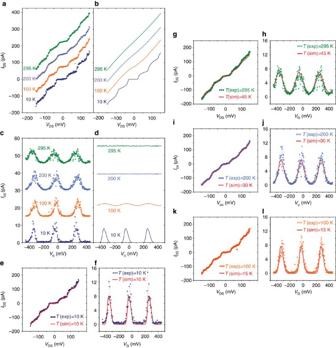Figure 5: Use of cold electrons in single-electron transistors (SETs). (a) MeasuredI–Vcharacteristics of a fabricated SET at different temperatures. The Coulomb staircase is clearly seen at all temperatures, including room temperature. Above 10 K, eachI–Vis vertically displaced by 75 pA from the lower temperature one for clarity.VDS: source-drain voltage.IDS: source-drain current. (b)I–Vcharacteristics calculated with orthodox theory under the usual Fermi-Dirac distribution (Simulator: SIMON 2.0). (c) Measured Coulomb oscillations at different temperatures.VG: gate voltage.VDSwas 10 mV. Above 10 K, eachI–Vis vertically displaced by 15 pA from the lower temperature one for clarity. (d) Coulomb oscillations calculated with orthodox theory under the usual Fermi-Dirac distribution. All temperatures indicated ina–dare the reservoir temperatures. (e,f) Comparison of the experimental and simulated Coulomb staircases (e) and Coulomb oscillations (f) at 10 K.T(exp): the reservoir temperature at which the experiment was carried out.T(sim): the simulation temperature. (g–l) Comparison of experimental and simulated Coulomb staircases and Coulomb oscillations at elevated reservoir temperatures (100–295 K). For the simulations, the effective electron temperatures were used in the orthodox theory calculation. Just a single set of parameters (except for the background chargeQ0) was used for all simulations inb,dande–l. The parameters areC1=0.85 aF,C2=2.9 aF,CG=0.52 aF,R1=8.7 × 107Ω andR2=6.6 × 108Ω. The background chargesQ0fore,f,g,h,i,j,kandlare −0.075e, 0.45e, 0.075e, 0.40e, −0.075e, 0.50e, −0.025eand 0.50e, respectively. Figure 5a,c display measured I – V characteristics of a fabricated SET at different temperatures. Over all temperatures studies, including room temperature, we observe clear single-electron transport behaviour, that is, Coulomb staircases ( Fig. 5a ) and Coulomb oscillations ( Fig. 5c ). The SET characteristics at higher temperatures, 100–295 K, highlight the effectiveness of our method as follows. First, we note that at the lowest temperature (10 K) the Coulomb staircase and Coulomb oscillations are accurately described by the orthodox theory of single-electron transport [3] , [50] ( Fig. 5e–f ). Now, we see that these low-temperature SET characteristics are well preserved even at much higher temperatures (100–295 K; Fig. 5a,c ). We note that with the usual Fermi-Dirac thermal smearing in effect (that is, no energy filtering), the Coulomb staircases and Coulomb oscillations are substantially or completely wiped out at these temperatures ( Fig. 5b,d ). Figure 5: Use of cold electrons in single-electron transistors (SETs). ( a ) Measured I–V characteristics of a fabricated SET at different temperatures. The Coulomb staircase is clearly seen at all temperatures, including room temperature. Above 10 K, each I – V is vertically displaced by 75 pA from the lower temperature one for clarity. V DS : source-drain voltage. I DS : source-drain current. ( b ) I – V characteristics calculated with orthodox theory under the usual Fermi-Dirac distribution (Simulator: SIMON 2.0). ( c ) Measured Coulomb oscillations at different temperatures. V G : gate voltage. V DS was 10 mV. Above 10 K, each I – V is vertically displaced by 15 pA from the lower temperature one for clarity. ( d ) Coulomb oscillations calculated with orthodox theory under the usual Fermi-Dirac distribution. All temperatures indicated in a – d are the reservoir temperatures. ( e,f ) Comparison of the experimental and simulated Coulomb staircases ( e ) and Coulomb oscillations ( f ) at 10 K. T (exp): the reservoir temperature at which the experiment was carried out. T (sim): the simulation temperature. ( g – l ) Comparison of experimental and simulated Coulomb staircases and Coulomb oscillations at elevated reservoir temperatures (100–295 K). For the simulations, the effective electron temperatures were used in the orthodox theory calculation. Just a single set of parameters (except for the background charge Q 0 ) was used for all simulations in b , d and e – l . The parameters are C 1 =0.85 aF, C 2 =2.9 aF, C G =0.52 aF, R 1 =8.7 × 10 7 Ω and R 2 =6.6 × 10 8 Ω. The background charges Q 0 for e , f , g , h , i , j , k and l are −0.075 e , 0.45 e , 0.075 e , 0.40 e , −0.075 e , 0.50 e , −0.025 e and 0.50 e , respectively. Full size image The preservation of the Coulomb staircases and Coulomb oscillations at elevated reservoir temperatures is explained by the fact that the energy-filtered electrons are much colder than the reservoir. Effective electron temperatures of energy-filtered electrons are ~45, ~30 and ~15 K for the reservoir temperatures 295, 200 and 100 K, respectively (from Fig. 3d and equation (6) in Supplementary Note 4 ). These low electron temperatures explain the experimental data in Fig. 5a,c extremely well. This is shown in Fig. 5g–l , in which the orthodox theory calculations (red lines) at these low temperatures faithfully reproduce all the experimental Coulomb staircase and Coulomb oscillation data. The benefit of having low-temperature electrons is clear in the current SET example: the requirement of liquid He cooling can be lifted, yet the low-temperature SET performance remains. With similar methodology, it is highly probable that the same benefit can be extended to other systems, such as spintronic and optoelectronic devices. It is worthwhile here to highlight one important element that has enabled the room-temperature energy filtering of the present study. It is the large separation between quantum levels in the QW energy filter. For energy filtering through a quantum state to work at room temperature, the level spacing between adjacent quantum levels in the energy filter must be appreciably larger than room-temperature thermal energy, ~25 meV. The narrow quantum confinement in the QW layer is able to produce large energy level separations because a QW can reliably be made very thin, a few nm’s. For the chromium oxide QW of the present study, its thickness (~2 nm) along with its QW depth (~1 eV) produces energy level spacing larger than 250 meV ( Supplementary Figs 2, 9 and Supplementary Notes 1, 6 ). This level separation is more than ten times larger than room-temperature thermal energy, making room-temperature energy filtering possible. An added practical benefit of the QW energy filter is its facile formation. For the chromium oxide QW we used, the oxide is spontaneously formed on the chromium electrode surface, a relatively simple and controllable procedure. In addition, the materials used in the QW energy filter formation (for example, Cr, Cr 2 O 3 and SiO 2 ) are compatible with mainstream CMOS materials and processes. This CMOS compatibility is an attribute that is likely to encourage development of the present energy filtering method for practical device applications. For future research, it is instructive to identify key elements that would enable lowering electron temperature even further and make the energy-filtered cold electron transport more powerful. In principle, if there is no nearby energy state in the QW to which the electron can be thermally excited, the tunnelling of an electron from the source electrode to the QW state leaves the electron at zero temperature [9] , [10] . Furthermore, if the electron does not gain energy during the subsequent tunnelling event to the QD, the electron temperature would remain effectively at zero Kelvin. If these two conditions were fulfilled, we may envision electron transport at extremely low electron temperatures. The first condition can be satisfied relatively easily as the energy level separation in the QW can be made much larger than the room temperature thermal energy [17] , [24] (see also Supplementary Note 6 ). Fulfilling the second condition, that is, blocking energy-gaining pathways, however, is not straightforward and would need more detailed studies. Phonon absorption, for example, would depend on many factors including the effective Debye cutoff frequency, materials used (QD, dielectric, passivation layers, etc. ), device dimensions (for example, QD size) and geometric configuration. Understanding these factors and engineering them could enable more effective blocking of energy-gaining pathways, which would result in much colder electrons than those in the present study. How to cite this article : Bhadrachalam, P. et al . Energy-filtered cold electron transport at room temperature. Nat. Commun . 5:4745 doi: 10.1038/5745 (2014).